Gate-tuned normal and superconducting transport at the surface of a topological insulator Three-dimensional topological insulators are characterized by the presence of a bandgap in their bulk and gapless Dirac fermions at their surfaces. New physical phenomena originating from the presence of the Dirac fermions are predicted to occur, and to be experimentally accessible via transport measurements in suitably designed electronic devices. Here we study transport through superconducting junctions fabricated on thin Bi 2 Se 3 single crystals, equipped with a gate electrode. In the presence of perpendicular magnetic field B, sweeping the gate voltage enables us to observe the filling of the Dirac fermion Landau levels, whose character evolves continuously from electron- to hole-like. When B =0, a supercurrent appears, whose magnitude can be gate tuned, and is minimum at the charge neutrality point determined from the Landau level filling. Our results demonstrate how gated nano-electronic devices give control over normal and superconducting transport of Dirac fermions at an individual surface of a three-dimensional topological insulators. The classification of crystalline solids in terms of their electronic properties as metals and insulators is one of the early successes of quantum mechanics. Metals are those materials in which a finite density of states at the Fermi energy enables electrons to move freely, and to conduct electricity. On the contrary, when the Fermi energy lies in an energy gap with no electronic state available, electrons cannot propagate, causing the insulating behaviour. Remarkably, it has been recently discovered [1] , [2] that this long-established classification is incomplete: topological insulators (TIs), realized in compounds with very strong spin–orbit interaction, represent a third class of materials, possessing an energy gap in their bulk—similarly to insulators—and electronic states that remain ungapped—such as in a metal—at their surfaces. The nature of the surface states in TIs depends on their dimensionality. In two-dimensional (2-D) TIs, they consist of one-dimensional helical modes propagating at the system edges [1] , [2] , whose existence has been revealed in transport experiments [3] , [4] . In the three-dimensional (3-D) case, the surface states are 2-D gases of Dirac fermions [5] , [6] , [7] , [8] , [9] . Following theoretical predictions [6] , [9] , Dirac fermions have been observed in several bismuth-based materials in angle-resolved photoemission experiments [10] , [11] , [12] and scanning tunnelling spectroscopy [13] , [14] . Contrary to the 2-D case, however, for 3-D TIs probing and controlling Dirac fermions in transport measurements [15] , [16] , [17] , [18] , [19] is difficult, because a large parallel conductance originating from bulk states is usually present [18] , [20] , [21] , [22] , [23] . This hinders the use of nano-fabricated devices based on 3-D TIs, which is essential to gain control over the Dirac fermions and to probe some of their most unique properties. Here we study transport through thin (~10 nm) Bi 2 Se 3 layers exfoliated from single crystals and transferred onto (doped) Si/SiO 2 substrates functioning as gates, and we show that the ability to modulate the carrier density is a powerful tool to investigate Dirac surface fermions. As superconductor/TI junctions are of interest for the investigation of so-called Majorana fermions [24] , [25] , the Bi 2 Se 3 layers were contacted with two closely separated Al/Ti superconducting electrodes ( T c ~1 K; Fig. 1 ), enabling us to investigate in a same device the normal state transport at high magnetic field B , and the possibility to gate-control induced superconductivity at B =0. 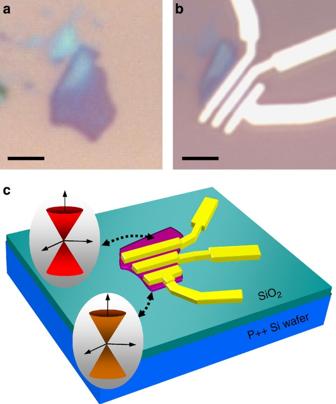Figure 1: Electrostatically gated devices based on a 3-D TI. (a) Optical microscope image of a thin layer of Bi2Se3on a Si/SiO2substrate, produced by exfoliation of a single crystal. The thickness is estimated to be ~10 nm, from measurements carried out with a Keyence microscope equipped with a laser interferometer. (b) Optical microscope image of the same layer with three Al/Ti (75/5 nm) contacts, forming two superconducting junctions. The contact separationLis ~400 nm; the widthWof the two junctions is ~3.2 and 2 μm, respectively, (all data shown in this paper have been obtained from the junction formed between the central and the left electrode; the other junction shows an essentially identical behavior). Scale bar, 2 μm. (c) Schematic representation of the complete device, with the degenerately doped silicon wafer functioning as a gate (the SiO2thickness is ~300 nm). A family of Dirac fermions resides on each surface of the Bi2Se3layers, represented by the so-called Dirac cones. Figure 1: Electrostatically gated devices based on a 3-D TI. ( a ) Optical microscope image of a thin layer of Bi 2 Se 3 on a Si/SiO 2 substrate, produced by exfoliation of a single crystal. The thickness is estimated to be ~10 nm, from measurements carried out with a Keyence microscope equipped with a laser interferometer. ( b ) Optical microscope image of the same layer with three Al/Ti (75/5 nm) contacts, forming two superconducting junctions. The contact separation L is ~400 nm; the width W of the two junctions is ~3.2 and 2 μm, respectively, (all data shown in this paper have been obtained from the junction formed between the central and the left electrode; the other junction shows an essentially identical behavior). Scale bar, 2 μm. ( c ) Schematic representation of the complete device, with the degenerately doped silicon wafer functioning as a gate (the SiO 2 thickness is ~300 nm). A family of Dirac fermions resides on each surface of the Bi 2 Se 3 layers, represented by the so-called Dirac cones. Full size image Gate-tuned Shubnikov-de Haas oscillations of Dirac fermions We realized several similar devices and here we discuss data measured on one of them that are representative of the overall behaviour observed (data from the other devices are shown in Supplementary Note 1 ). We first discuss the dependence of the normal state resistance measured at T= 4.2 K on gate voltage V g and magnetic field B , focusing on the qualitative aspects of the data, which are sufficient to conclude that Dirac surface fermions are present and can be gate controlled. The sample resistance is R =70 Ω and shows a 15–20% variation when V g is swept from −80 V to +50 V, roughly symmetrical with respect to V g CN ~−10 V ( Fig. 2a ). This non-monotonic dependence is a manifestation of ambipolar transport involving both electrons and holes, and indicates that the Fermi level at the Bi 2 Se 3 surface is located in the gap between valence and conduction bulk bands [26] , [27] . 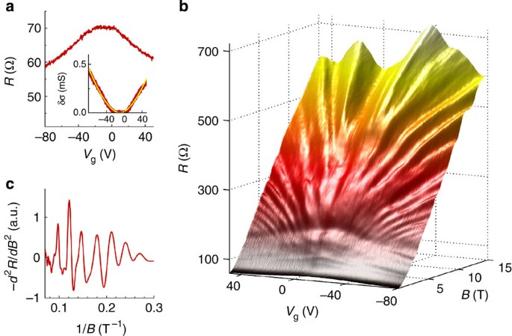Figure 2: Gate voltage and magnetic field dependence of the normal state resistance. (a) Gate voltage dependence of the normal state resistance. The maximum atVg~−10 V, provides a first indication of ambipolar transport. TheVgdependence originates from the modulation of the conductivity of the surface close to the gate, and can be quantitatively described asδσ(Vg)=nDirac(Vg)eμ(nDirac(Vg) is given by equation (1) withμ=2500 cm2Vs−1(inset of panel (a): the yellow line corresponds to the calculated δσ(Vg)). (b) Full dependence of the resistance onVgand magnetic fieldB(the measurements are performed by sweepingVgat fixedB, for different values ofB). As a function ofBthe resistance increases approximately linearly, exhibiting clear oscillations that are enhanced by deriving the data with respect to eitherVgorB. (c) Oscillations in −d2R/dB2(Vg=−62 V), periodic in1/Bas it is typical for the SdH effect (for small oscillations superimposed on a slowly varying background −d2R/dB2has the same phase as the oscillations in the resistance itself). All data shown in this figure were measured at 4.2 K. Figure 2: Gate voltage and magnetic field dependence of the normal state resistance. ( a ) Gate voltage dependence of the normal state resistance. The maximum at V g ~−10 V, provides a first indication of ambipolar transport. The V g dependence originates from the modulation of the conductivity of the surface close to the gate, and can be quantitatively described as δ σ( V g )= n Dirac ( V g ) eμ ( n Dirac ( V g ) is given by equation (1) with μ =2500 cm 2 Vs −1 (inset of panel ( a ): the yellow line corresponds to the calculated δσ( V g )). ( b ) Full dependence of the resistance on V g and magnetic field B (the measurements are performed by sweeping V g at fixed B , for different values of B ). As a function of B the resistance increases approximately linearly, exhibiting clear oscillations that are enhanced by deriving the data with respect to either V g or B . ( c ) Oscillations in − d 2 R / dB 2 ( V g =−62 V), periodic in 1/B as it is typical for the SdH effect (for small oscillations superimposed on a slowly varying background − d 2 R / dB 2 has the same phase as the oscillations in the resistance itself). All data shown in this figure were measured at 4.2 K. Full size image With increasing B , the resistance also increases, reaching values close to 1 k Ω at 15 T ( Fig. 2b ). Oscillations periodic in 1/B are clearly visible ( Fig. 2c ), as it is characteristic for the Shubnikov-de Haas (SdH) effect [28] ( Fig. 2b ). The oscillations are gate-voltage-dependent and disperse in opposite directions when V g is swept across V g CN , which indicates that the character of the charge carriers changes from electron ( V g > V g CN ) to hole ( V g < V g CN ). These oscillations are not present when the magnetic field is applied parallel to the surface of the Bi 2 Se 3 flake ( Supplementary Note 2 ). Additional information can be obtained if the amplitude of the oscillations is enhanced by looking at the quantities − d 2 R / dB 2 ( B , V g ) and − d 2 R / dV g 2 ( B , V g ) ( Fig. 3a,b respectively) or by subtracting the positive magnetoresistance background ( Supplementary Note 3 ). The two methods give fully consistent results, and here we focus on the discussion of the second derivative, which is free from any possible arbitrariness associated to the background subtraction. 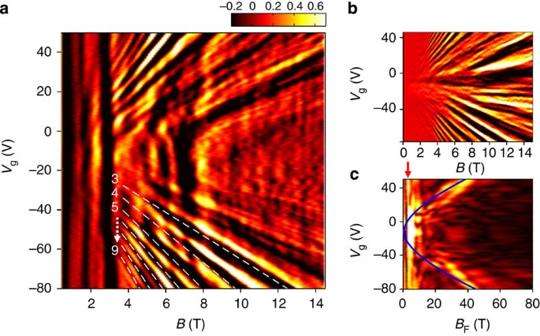Figure 3: Fan diagram of Landau levels of Dirac electrons and holes. (a) Plot of −d2R/dB2(in arbitrary units) as a function ofBandVg(fan diagram). The features dispersing withVgoriginate from the formation of Landau levels of Dirac fermions on the bottom surface of the Bi2Se3crystal. Features with aVg-independent position are associated to Landau levels on the top surface. The white dashed lines (and the numbers indexing the LLs) indicate the condition for the Fermi level to fall between two Landau levels for holes on the bottom surface (seediscussionin the main text). They correspond to(nis the density of Dirac holes), as expected for Dirac fermions. A similar indexing also works for electrons (i.e., positive gate voltage). (b) −d2R/dVg2plot showing dispersing features corresponding to those observed in the −d2R/dB2plot (theVg-independent features disappear when taking theVgderivative). An asymmetry between electrons and holes at high magnetic field—already visible in the—d2R/dB2plot—is present, which is likely to originate from the opening of a small Zeeman gap16, which shifts the position of the zero-energy LL to either positive or negative energies depending on the sign of theg-factor. (c) Fourier spectrum of −d2R/dB2, as a function ofVgand frequencyBF. From the position maxima in the spectrum we extract the density of carriers according to the relationn=BFe/h. Again, the features dispersing withVgoriginate from Landau levels of Dirac fermions on the bottom surface, and theVg-independent features (pointed to by the red arrow), from states on the top surface. AtVg=0 V, the peaks of the dispersing and non-dispersing features occur approximately at the same frequency, implying that the density of electrons on the two surfaces of the crystal are also the same. The blue line is the frequency of the SdH oscillations calculated using equation (1) (BF=nDirac(Vg)h/e) with no free parameter, in good agreement with the gate dependent position of the (broad) peak in the Fourier spectrum. Figure 3a shows that—next to the oscillations dispersing with V g —features that do not depend on gate voltage are also present. These features are also periodic in 1/B : indeed the Fourier spectrum of the data plotted versus 1/B ( Fig. 3c ) shows a peak dispersing with gate voltage as well as a peak whose position is V g -independent. Interestingly, at V g =0 V the frequency of the two peaks—the one dispersing with gate voltage and the V g —independent one—are nearly the same. Figure 3: Fan diagram of Landau levels of Dirac electrons and holes. ( a ) Plot of − d 2 R / dB 2 (in arbitrary units) as a function of B and V g (fan diagram). The features dispersing with V g originate from the formation of Landau levels of Dirac fermions on the bottom surface of the Bi 2 Se 3 crystal. Features with a V g -independent position are associated to Landau levels on the top surface. The white dashed lines (and the numbers indexing the LLs) indicate the condition for the Fermi level to fall between two Landau levels for holes on the bottom surface (see discussion in the main text). They correspond to ( n is the density of Dirac holes), as expected for Dirac fermions. A similar indexing also works for electrons (i.e., positive gate voltage). ( b ) − d 2 R / dV g 2 plot showing dispersing features corresponding to those observed in the − d 2 R / dB 2 plot (the V g -independent features disappear when taking the V g derivative). An asymmetry between electrons and holes at high magnetic field—already visible in the— d 2 R / dB 2 plot—is present, which is likely to originate from the opening of a small Zeeman gap [16] , which shifts the position of the zero-energy LL to either positive or negative energies depending on the sign of the g -factor. ( c ) Fourier spectrum of − d 2 R / dB 2 , as a function of V g and frequency B F . From the position maxima in the spectrum we extract the density of carriers according to the relation n = B F e/h . Again, the features dispersing with V g originate from Landau levels of Dirac fermions on the bottom surface, and the V g -independent features (pointed to by the red arrow), from states on the top surface. At V g =0 V, the peaks of the dispersing and non-dispersing features occur approximately at the same frequency, implying that the density of electrons on the two surfaces of the crystal are also the same. The blue line is the frequency of the SdH oscillations calculated using equation (1) ( B F =n Dirac (V g )h/e ) with no free parameter, in good agreement with the gate dependent position of the (broad) peak in the Fourier spectrum. Full size image These observations give clear indications as to the nature of the electronic states that are involved. Finding an electron-to-hole crossover that occurs in a small gate voltage range (~10 V) —which corresponds to a rather small amount of accumulated charge (few times 10 11 cm −2 )—implies that the electronic states responsible for the SdH oscillations cannot be in the bulk band of the material. As the bulk bands are separated by a gap of ~300 meV [12] , crossing over from electron to holes would require a change in gate voltage that is well more than one order of magnitude larger. A continuous crossover from electron to hole SdH is known to occur (and has been observed) only in gapless systems of chiral fermions (for example, graphene or bilayer graphene [29] ). Indeed gapless Dirac fermions are known to be present at the surface of Bi 2 Se 3 (refs 19 , 12 , 13 , 14 ). The electron-to-hole crossover as a function of gate voltage that we observe in the SdH oscillations, therefore, is a clear indication of the presence of Dirac fermions in our devices. It also confirms, as it was already concluded from the observation of ambipolar transport at B=0 T, that the Fermi level at the surface is inside the gap of the bulk bands of Bi 2 Se 3 . The conclusion that Dirac fermions are responsible for the V g -dependent SdH oscillations also explains the presence of SdH oscillations with a V g -independent frequency. In fact, Dirac fermions are not only present on the bottom surface of the Bi 2 Se 3 flake but also on the top surface. As this top surface is further away from the gate electrode, it is electrostatically screened by carriers that are accumulated on the bottom surface and by states that are present in the 'bulk' of the flake (see below). Accordingly, sweeping the gate voltage does not lead to a change in the carrier density on the top surface, and the frequency of the SdH oscillations associated to these carriers is constant. The finding that at V g =0 V, the V g -independent and the V g -dispersing oscillations have roughly the same frequency can be explained naturally, as when no gate voltage is applied the two surfaces of the Bi 2 Se 3 flake host approximately the same carrier density. This finding could not be explained if the two families of SdH oscillations had different origin. We conclude that the presence of surface Dirac fermions at the surface of Bi 2 Se 3 explains all the qualitative aspects of our observations—continuous evolution from electron to hole SdH, the presence of two families of SdH with different response to the gate voltage and having the same frequency at V g =0 V, and the observation of ambipolar transport. No other known scenario can account for these findings. Bulk contribution to the magnetoresistance Having established the presence of Dirac surface fermions from qualitative aspects of the data only is important, because it ensures that this conclusion does not depend on any specific assumption that needs to be made to interpret detailed aspects of the data quantitatively. To proceed with such a more quantitative analysis, we first note that in our devices another transport channel in parallel to the surface states is present, which gives a dominant contribution to the measured conductance. Indeed, the device resistance—approximately 70 Ω—is much smaller than what can be expected from the presence of surface Dirac fermions alone. To estimate the conductivity of Dirac fermions, a carrier mobility μ of 1000–2000 cm 2 Vs −1 can be taken, corresponding to the best values reported in the literature for Bi 2 Se 3 (refs 26 , 27 ; see also below). We then find that, at high gate voltage, the parallel conductivity is almost 10 times larger than the surface conductivity ( Supplementary Note 4 ). The surface Dirac states therefore coexist with other states in the system present inside the Bi 2 Se 3 flake, at the same energy (that is, inside the gap between bulk conduction and valence band). We attribute the origin of these states to the presence of an impurity band [21] caused by the disorder present in Bi 2 Se 3 , which is known to be large even in the best crystals. Indeed, a rather large density of states inside the gap, coexisting with the surface Dirac fermion states, is reproducibly seen in scanning tunnelling spectroscopy experiments [14] , [30] . The density of states ν Bulk coexisting with the Dirac surface states can be estimated by comparing the density of charge extracted from the SdH frequency B F with that obtained from the known capacitance to the gate voltage. At V g − V g CN =−70 V, for instance, the frequency of the SdH oscillations corresponds to a density n=B F e/h =1.05×10 16 m −2 , whereas C(V g − V g CN )=5.1×10 16 m −2 . The discrepancy is only apparent, because with changing V g charge is accumulated near the surface on a depth given by the Thomas–Fermi screening length ( λ TF ~3–4 nm) and the occupation of states in the impurity band reduces the density of Dirac fermions n Dirac ( V g ) to (only a fraction of the accumulated charge occupies Dirac fermion states): with n Tot = C | V g − V g CN |/ e and ν F =5 10 5 m/s ( Supplementary Note 5 ). By imposing that at V g =−80 V n Dirac ( V g ) coincides with the density extracted from the fan diagram, we obtain ν Bulk λ TF =3.6 10 13 cm −2 eV −1 , corresponding to ν Bulk ~7 10 19 cm −3 eV −1 , comparable to literature estimates for similar crystals [21] . We can then use equation (1) to calculate the frequency of the SdH oscillations for all values of V g , B F ( V g )=( h / e ) n Dirac ( V g ), and we find quantitative agreement with the position of the peak in the Fourier spectrum with no adjustable parameters (blue line in Fig. 3c ). Equation (1) also naturally reproduces the V g dependence of the conductivity ( δ σ( V g )) at B =0. The inset of Fig. 2a shows that δ σ( V g )= n Dirac ( V g ) eμ is in excellent agreement with the measured data with μ =2500 cm 2 Vs −1 . This value is comparable, but slightly higher, than what has been reported previously for Bi 2 Se 3 surface states [26] , [27] ; when inserted in the criterion for the occurrence of SdH oscillations, ω c τ = μB ≥1 (ref. 28 ), it gives B ≥4T, which agrees with experiments (oscillations due to top-surface Dirac electrons start at approximately half this field—implying μ ~5000 cm 2 Vs −1 —probably because contact with SiO 2 slightly reduces μ at the bottom surface). Landau levels for Dirac fermions We now proceed to discuss the indexing of the Landau levels responsible for the SdH. For massless Dirac fermions, when n=(N+1/2) B/(h/e) , the N th LL is completely filled and the Fermi energy is located in between the N th and the ( N+1) th LLs (here n is the density of surface Dirac fermions, N the integer LL index and B/(h/e) is the LL degeneracy [29] ). A quantitative interpretation of the data measured in our samples, however, requires an assumption to be made: it is a priori unclear whether maxima or minima of the measured oscillations correspond to having completely filled LLs at the surface, because both conductance of the Dirac fermions and parallel conductance depends on magnetic field. As the background conductance is 10× larger than the conductance of the surface states, its contribution to the oscillations is likely to dominate. We therefore assume that the dominant contribution to the magnetoresistance oscillations is due to the background conductance itself, which is modulated by the formation of surface LLs. Specifically, with the flake being only 10 nm thick, carriers responsible for the background conductance are strongly coupled to the surface states (this is indicated by the fact that the diffusion constant of these carriers and of the Dirac surface fermions is approximately the same, as discussed in Supplementary Note 4 ). When the Fermi level at the surface is inside (in between) LLs, the density of states at the Fermi energy associated to the surface LLs has a maximum (minimum), so that carriers responsible for the background conductance have maximum (minimum) probability to scatter, and the background resistance is also maximum (minimum; in other words, the formation of surface LLs modulates the diffusion constant of the carriers responsible for the background conductance). On this basis, we index the LLs by taking resistance minima in the oscillations (as illustrated by the white dashed lines in Fig. 3a ) and plot the index N as a function of 1/B . For massless Dirac fermions , that is, the LL index N scales linearly with 1/ B , and extrapolates to −1/2 for . The analysis of the value of N extrapolated from the actual data through a linear fit is shown in Fig. 4 , for all values of gate voltage for which the quality of the SdH oscillations is sufficient to perform the quantitative analysis ( V g between −80 and −40 V for holes and between +15 and +50 V for electrons). For the different values of V g , we find that the extrapolation b indeed fluctuates close to −0.5, and the average of b over the entire gate voltage range is ‹ b ›=−0.4±0.1 as expected for massless Dirac fermions [29] . Despite requiring an assumption (that is, that the oscillations are dominated by the conductance in parallel to that of the Dirac fermion states), this analysis is important because it shows that a simple physical scenario exists that is based on what has been established about our system (presence of surface Dirac fermions and of a large parallel conductance) and is capable of accounting for our observations quantitatively, in an internally consistent way. 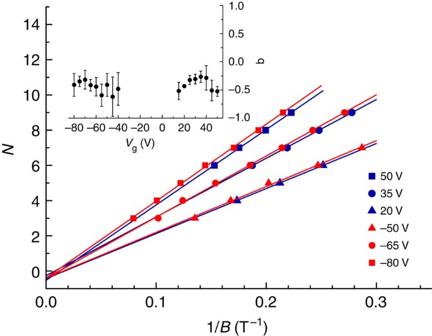Figure 4: Massless Dirac character of surface fermions. Main panel: Landau level indexNversus1/Bplotted for selected values of gate voltage, corresponding to different concentrations of holes (red symbols) and electrons (blue symbols). According to the relation characteristic for massless Dirac fermions,, wherenis the density of charge carriers (electrons or holes), whereas for normal fermions. Therefore, looking at howNextrapolates forallows us to discriminate between massless Dirac and normal fermions. The continuous lines are linear least square fits to the data. They show that as,Nextrapolates to close to−1/2as expected for massless Dirac fermions. The inset shows the extrapolation value (b) obtained by least square fitting for ~20 different values of gate voltage (in the region with Vg in between ~−40 and +15 V, the oscillations are not sufficiently pronounced to perform the analysis). The data show thatbfluctuates close to−1/2(and not around0). Consistently, the average ofbover gate voltage is ‹b›=−0.4±0.1. Figure 4: Massless Dirac character of surface fermions. Main panel: Landau level index N versus 1/B plotted for selected values of gate voltage, corresponding to different concentrations of holes (red symbols) and electrons (blue symbols). According to the relation characteristic for massless Dirac fermions, , where n is the density of charge carriers (electrons or holes), whereas for normal fermions . Therefore, looking at how N extrapolates for allows us to discriminate between massless Dirac and normal fermions. The continuous lines are linear least square fits to the data . They show that as , N extrapolates to close to −1/2 as expected for massless Dirac fermions. The inset shows the extrapolation value ( b ) obtained by least square fitting for ~20 different values of gate voltage (in the region with Vg in between ~−40 and +15 V, the oscillations are not sufficiently pronounced to perform the analysis). The data show that b fluctuates close to −1/2 (and not around 0 ). Consistently, the average of b over gate voltage is ‹ b ›=−0.4±0.1. Full size image Gate-tuned supercurrent through surface states Measurements at B =0 and T =30 mK, with the Al/Ti electrodes in the superconducting state ( T c ~1 K), show that the ability to gate-control the device is also essential to establish that the Dirac fermions contribute to mediate the superconducting correlations induced by the contacts. In the measured differential resistance, a large suppression is observed when the bias is decreased below twice the superconducting gap ( Fig. 5a ), a distinctive signature of Andreev reflection, indicating the high transparency of the contacts [31] . At zero bias, a supercurrent is present ( Fig. 5b ), with critical current I c ~200 nA. It is apparent that the critical current depends on the gate voltage, and that it has a minimum in correspondence of the charge neutrality point extracted from the LL fan diagram. This finding shows the ambipolar character of the supercurrent, and makes clear directly from the experimental data that at least part of the supercurrent is carried by either Dirac electrons or holes at the bottom Bi 2 Se 3 surface (and not only by the carriers in the bulk states). By enabling to separate the contributions of the surface and bulk channels to superconducting transport, gate control of supercurrent certainly provides an effective tool for the investigation of proximity effect in 3-D TIs (whose complete understanding—for example, the very small R n I c product, ~15 μV<<2Δ /e ~300 μV— Fig. 5c —goes beyond the scope of this paper). 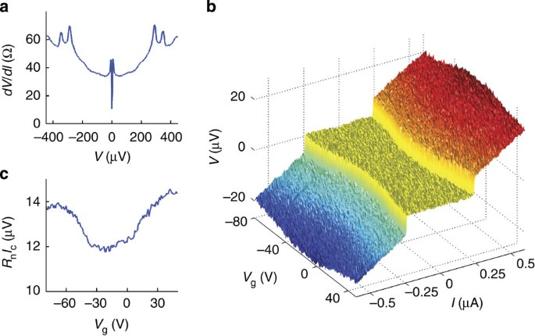Figure 5: Gate-tunable supercurrent. (a) Differential resistance of the junction in the superconducting state (B=0,T=30 mK), as a function of bias voltageV(Vg=+50 V). A large decrease is seen upon loweringVbelow 2Δ/e~300 μeV, due to Andreev reflection (the sharp feature aroundV=0 originates from the presence of the supercurrent; the origin of the split peak atV~2Δ/eis currently unknown). (b) JunctionI-Vcurves showing a gate-tunable supercurrent. The critical current exhibits a minimum atVg~−10 V, corresponding to theVgvalue at which the maximum of the normal state resistance occurs. (c)RnIcproduct of the junction obtained using forRnthe measured normal state resistance. Its value (~15 μeV) is about 20 times smaller than expected (RnIc~2Δ/e~300 μeV). Figure 5: Gate-tunable supercurrent. ( a ) Differential resistance of the junction in the superconducting state ( B =0, T =30 mK), as a function of bias voltage V ( V g =+50 V). A large decrease is seen upon lowering V below 2Δ /e ~300 μeV, due to Andreev reflection (the sharp feature around V =0 originates from the presence of the supercurrent; the origin of the split peak at V ~2Δ /e is currently unknown). ( b ) Junction I-V curves showing a gate-tunable supercurrent. The critical current exhibits a minimum at V g ~−10 V, corresponding to the V g value at which the maximum of the normal state resistance occurs. ( c ) R n I c product of the junction obtained using for R n the measured normal state resistance. Its value (~15 μeV) is about 20 times smaller than expected ( R n I c ~2Δ/ e ~300 μeV). Full size image Our experiments clearly show how the use of a gate electrode to tune the surface density of charge carriers is a very effective tool to identify and explore the contribution to transport of surface Dirac fermions in devices based on 3-D TIs. The possibility to tune the carrier density electrostatically, for instance, enables the observation of Dirac electron and hole transport in a single device, making it possible to control the filling of their Landau levels. It also allows the identification of transport properties associated with the two opposite material surfaces, owing to their different electrostatic coupling to the gate electrode. Finally, it is crucial to establish that Dirac fermions are capable of mediating superconducting correlations induced by the contacts, a conclusion drawn directly from the experimental data that—in the presence of a large parallel contribution to transport—would be difficult to draw in any other way. It appears from our experiments that the quality of the BiSe-based 3-D topological materials currently available would greatly benefit from considerable improvements, which should aim at decreasing the amount of states present in the bulk bandgap of the crystals and at increasing the carrier mobility. Nevertheless, even with the quality of the existing materials, performing new and interesting transport experiments, to investigate the physics of Dirac surface fermions is certainly possible. These experiments should address, among other, the detailed behaviour of the Dirac fermions as a function of the crystal thickness [32] , [33] —where ARPES experiments have shown an interesting dimensional crossover to occur [34] —and the nature of proximity effect [24] , [25] , both of which currently remain phenomena virtually unexplored experimentally. Growth of Bi 2 Se 3 single crystals Single crystals of Bi 2 Se 3 were grown by a floating zone method. Bismuth and selenium were weighted in stoichiometric ratio and sealed under vacuum (~10 −3 mbar) in quartz ampoules. According to the Bi–Se phase diagram, Bi 2 Se 3 has a congruent melting point at 705 °C [35] . To synthesize the compound, the mixture of elements was heated up to 750 °C, kept at this temperature for 12 h and then quenched to room temperature. To assure a better mixing of the elements, during the isothermal time in the liquid state, the ampoule was shaken and rotated. This procedure was repeated three times. Finally the ampoule was heated up to 820 °C for 24 h and slowly cooled down to room temperature. At the end of this procedure, the sample was already formed by large single domains of good quality, suggesting a high growth rate for Bi 2 Se 3 . The sample was then crushed into small pieces and sealed inside a quartz ampoule with 5 mm of inner diameter and a conical bottom, which was vertically mounted in a homemade 2-lamp furnace. The sample was moved downwards through the hot zone at a speed of ~0.33 mm h −1 , starting from the apex of the conical tip. In this way a single crystal started to grow in the tip. The ampoule was kept rotating all the time to avoid lateral thermal gradient. The advantage of the floating zone over other growth techniques consists in the large temperature gradient at the growth interface, the low travelling velocity, and the fact that the growing composition is prevented from local fluctuations in the melt composition. These differences can account for a different structural quality of the crystals—and in particular a lower density of defects—as compared with that of existing materials grown by different techniques. Large (1–10 mm size) crystals were cleaved from the solid rod formed inside the quartz. The high crystalline quality of the crystals was confirmed by X-ray diffraction that shows a single phase, single index diffraction pattern and narrow rocking curves. The cell parameters were found to be in good agreement with those reported in the literature. Device fabrication Thin layers of Bi 2 Se 3 were obtained by exfoliation of single crystals using an adhesive tape, while monitoring the process under an optical microscope, similarly to what is carried out to extract graphene from graphite [36] . The layers were transferred onto a degenerately doped Si substrate (functioning as a gate electrode) covered with a 300-nm layer of thermally grown SiO 2 (gate insulator), simply by pressing the adhesive tape onto the substrate. Most layers produced in this way appeared to be shiny when observed under the microscope, corresponding to a large thickness (several tens of nanometres or more). In few cases, however, thinner layers (characterized by a darker colour) were also found (the thinnest layer that we observed had a thickness of approximately 4 nm). These thinner layers were selected for the fabrication of devices. Compared with graphene, producing very thin Bi 2 Se 3 layers is considerably more difficult because Bi 2 Se 3 is more brittle than graphite, and the material tends to easily break into very small pieces during the exfoliation process. Devices were fabricated by conventional nano-fabrication techniques: electron-beam lithography was used to generate the contact pattern, and electron-beam evaporation followed by lift-off was used to define the Al/Ti (75/5 nm) electrodes. Electrical measurements The devices were cooled down using either a Kelvinox 400 dilution refrigerator or a He3 insert, mounted into a cryostat equipped with a 15 T superconducting magnet, and measured in the range between 30 mK and 250 K. The dilution refrigerator contained copper powder filters at the mixing chamber stage, necessary to observe a finite supercurrent (all wires were also π-filtered at room temperature). The electrical characteristics were measured using a lock-in technique (magnetotransport), dc I-V curves (supercurrent measurements) or a combination of the two (bias dependent differential resistance measurements). The charge density in the devices was controlled by applying a gate voltage to the p-doped silicon substrate. Temperature dependence of the resistance As characterization of the Bi 2 Se 3 crystals used in our experiments, we have measured the temperature dependence (from 250 to 4.2 K) of the resistance for two devices fabricated as described in Section 2, and compared the results to measurements reported in the literature. The two devices were fabricated using nearby layers (~100 μm apart) found on a same substrate, implying that they originate from a same region of the starting bulk Bi 2 Se 3 crystal. The thickness of one of the layers was ~4 nm (as estimated using a Keyence microscope equipped with a laser interferometer) and that of the other was ~10 nm. The temperature dependence of the resistance is shown in Supplementary Figure S1 (unfortunately the 4-nm device broke early after starting the experiments). Although both layers were rather highly conducting ( ρ ~1 mΩ cm, in the range reported in the literature [20] , [21] , [22] , [23] ), the thinnest one was found to exhibit a weak insulating temperature dependence (resistance slightly increasing with lowering T ), whereas in the thicker one the resistance decreased with lowering T . This difference may indicate the opening of a gap in the surface states due to hybridization of the Dirac bands on opposite surfaces, which for a 4-nm thickness should lead to a gap of about 10 meV (for a 10-nm thickness the gap is predicted to be negligible). The large conductivity observed in nominally undoped Bi 2 Se 3 is usually attributed to the presence of unintentional electron doping [21] , which pins the Fermi level inside the bulk conduction band. Our gate-dependent studies, which exhibit the charge neutrality point at only approximately −10 V, show that our devices are also slightly electron doped. Nevertheless, the gate voltage dependence of the resistance also indicates that, contrary to what is most frequently reported in the literature [20] , [21] , [22] , [23] , in our thin layers, the Fermi level at the surface is not located in the bulk conduction band, but is located inside the gap. Note that from the Fourier transform of the SdH oscillations we can conclude that the density of surface carriers at V g =0 V is approximately the same on the two surfaces (see main text), implying that the Fermi level is inside the gap of the bulk bands also at the surface far away from the gate. As the Thomas–Fermi screening length is not much smaller than the thickness of the crystal, we conclude that the Fermi level is inside the gap throughout the thickness of our devices. Note that, even though the observed behaviour is different from that reported from studies of transport through bulk crystals, it is in line with the observation reported by Steinberg et al . [26] who studied transport through gated exfoliated flakes; their devices are comparable but somewhat thicker than ours—the thinnest flake reported in (ref. 26 ) is approximately 16 nm thick). As in our devices the Fermi level is located in the bulk gap, the electrical conductance that we measure is mediated by both the surface Dirac fermions, and by carriers occupying states in the impurity band inside the gap, whose presence is established in the literature. The impurity band originates from defect states with a large Bohr radius—about 4–5 nm, owing to the large relative dielectric constant of the material; ɛ~110 (ref. 21 ). This large radius causes a strong overlap of the impurity states, as well as a strong overlap of the impurity states with the surface Dirac fermion states (the Bohr radius of the impurity states is also comparable to the Bi 2 Se 3 layer thickness), resulting in a high conductivity in the impurity band. The large value of ɛ also suppresses Coulomb effects, which are usually the dominant mechanism lowering the conductivity of impurity bands, and tends to cause a more insulating-like behaviour through the opening of a Coulomb gap. Finally, note that the density of bulk impurity band states that we have extracted from the data, ν Bulk ~7×10 19 cm −3 eV −1 (see main text), is comparable to the density of states of the impurity band that forms in degenerately doped silicon. For silicon, an impurity band (that causes the material to be conducting at very low temperature) develops at doping concentrations of a 3–4×10 19 cm −3 (ref. 37 ). The states responsible for this impurity band are close to either the valence or the conduction band (depending on the sign of the dopants), and they are distributed in a fraction of 1 eV (corresponding to the gap of silicon). The resulting density of states (equal to the concentration divided by this energy range) coincides with the value that we estimated for Bi 2 Se 3 . As mentioned above, the conductivity in the impurity band is much larger in Bi 2 Se 3 as compared with silicon, because of the much larger dielectric constant, which suppresses Coulomb gap effects. How to cite this article: Sacépé B. et al . Gate-tuned normal and superconducting transport at the surface of a topological insulator. Nat. Commun. 2:575 doi: 10.1038/ncomms1586 (2011).